The stress-inducible ER chaperone GRP78/BiP is upregulated during SARS-CoV-2 infection and acts as a pro-viral protein 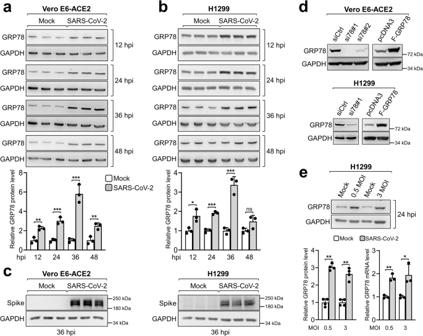Fig. 1: SARS-CoV-2 upregulated GRP78 protein and mRNA levels in infected cells. aVero E6-ACE2 cells were mock-infected or infected with SARS-CoV-2 at an MOI of 0.5 in triplicate. The cells were collected at 12, 24, 36, and 48 hr post infection (hpi) and cell lysates were analyzed by western blot for GRP78 protein level with GAPDH serving as loading control. Quantitation of relative protein level of GRP78 normalized against GAPDH was shown in the graph below (n= 3).bSame as inaexcept the human lung epithelial cell line H1299 was used (n= 3).cSame as inaandbbut 36 hpi cell lysates were analyzed by Western blot for SARS-CoV-2 Spike protein level with GAPDH serving as loading control (n= 3).dVero E6-ACE2 (upper) or H1299 (lower) cells were transiently transfected with control siRNA or siRNAs against GRP78 (left panel) or empty vector pcDNA3 or vector expressing full-length Flag-tagged GRP78 protein (F-GRP78) (right panel) for 48 hr. Cell lysates were analyzed by Western blot for GRP78 protein level with GAPDH serving as loading control.eH1299 cells were mock-infected or infected with SARS-CoV-2 at an MOI of 0.5 or 3. The cells were collected at 24 hpi and cell lysates were analyzed by western blot (n= 4) or RT-qPCR (n= 3) for GRP78 protein or mRNA levels, respectively, with GAPDH serving as an internal control. Quantitation of relative protein (left) or mRNA (right) levels of GRP78 normalized against GAPDH was shown in the graphs below. Data are means ± S.E.M. of three repeats. *P< 0.05; **P< 0.01; ***P< 0.001; ns denotes not significant (Student’sttest). Source data are provided as a Source Data file. 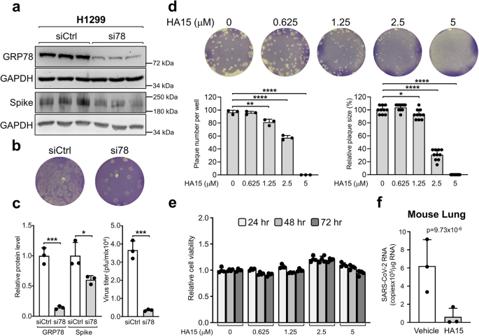Fig. 2: GRP78 knockdown by siRNA inhibited SARS-CoV-2 replication in vitro and GRP78 inhibitor HA15 blocked SARS-CoV-2 infection in vitro and in vivo. aH1299 cells were transiently transfected with control siRNA (siCtrl) or siRNA against GRP78 (si78#1) for 24 hr before infection with SARS-CoV-2 at an MOI of 3 for 24 hr. The cell lysates were analyzed by western blot for GRP78 and Spike protein levels with GAPDH serving as a loading control (n= 3).bThe supernatant containing the newly released virions fromawas collected and virus titer was determined by plaque assay (n= 3).cQuantitation of the relative protein levels of GRP78 and Spike normalized against GAPDH was shown in the graphs on the left and virus titer (pfu/ml) was shown in the graph on the right.dConfluent monolayers of Vero E6-ACE2 cells in six-well plates were infected with SARS-CoV-2 virus and treated with different concentrations of HA15 as indicated for 72 hr. At the end of treatment, the cells were stained with 0.2% crystal violet. The images are representatives of three repeats. Plaques were counted and plotted in the graph on the left (n= 3). Plaque size was measured and expressed relative to DMSO-treated control in the graph on the right (n= 10).eVero E6-ACE2 cells cultured under identical conditions as indwere treated with DMSO or increasing concentration of HA15 from 0.625 μM to 5 μM and cell viability was measured by WST-1 assay at 24, 48, and 72 hr after drug treatment (n= 4).fK18-hACE2 transgenic mice infected with SARS-CoV-2 were treated with vehicle control or HA15. Three days post infection, lung tissue RNA was isolated, and RT-qPCR was performed in triplicate reactions to detect SARS-CoV-2 N protein sequence (n= 3). Data are means ± S.E.M. of three repeats. *P< 0.05; **P< 0.01; ***P< 0.001; ****P< 0.0001 (Student’sttest). Source data are provided as a Source Data file. Cell culture and drug treatment The African green monkey kidney epithelial cell line Vero E6-ACE2 was cultured in Dulbecco’s modified Eagle medium (DMEM) containing 10% fetal bovine serum (FBS; Gemini Bio), 1% penicillin/streptomycin (pen/strep) (Corning Inc.), and 1 μg/ml puromycin. The human non-small cell lung adenocarcinoma cell line H1299 was cultured in RPMI-1640 medium containing 10% FBS and 1% pen/strep. All cell lines were maintained at 37 °C in a humidified atmosphere of 5% CO 2 and 95% air. HA15 was purchased from Sigma Aldrich and dissolved in DMSO. Vero E6-ACE2 cells were treated with HA15 at indicated concentrations and 1% DMSO was used as a control. The Vero E6 and H1299 cell lines were obtained from ATCC. Virus propagation The following reagent was deposited by the Centers for Disease Control and Prevention and obtained through BEI Resources, NIAID, NIH: SARS-Related Coronavirus 2, Isolate USA-WA1/2020, NR-52281. The virus was propagated in Vero E6-ACE2 in a DMEM media supplemented with 10% FBS, 1% penicillin-streptomycin (Gibco) and 0.5 µg/ml TPCK-treated trypsin (Worthington Biochemical). When 90% CPE was confirmed, supernatant was collected and passed through a 0.45 μm pore size polyethersulfone filter and aliquoted and stored at −80 °C until further use. The virus titer was determined by plaque assay. Plaque reduction assay Evaluating the anti-viral activities of HA15 was done by plaque reduction assay as described previously [18] . Confluent monolayers of Vero E6-ACE2 cells in 6-well plates were washed once with DMEM and infected with approximately 100 plaque-forming units (PFUs) of SARS-CoV-2 in each well. The plates were incubated in 33 °C for 45 min for virus adsorption. The virus inoculum was then removed and replaced by overlay media (DMEM containing 1% low-melting agarose without serum) containing 2-fold serial dilutions of HA15 and placed in 33 °C CO 2 incubator for 72 hr when plaques can be visualized under light. The cells were fixed with 4% formaldehyde solution for at least 30 min and the overlaid agarose was removed. The cells were stained with 0.2% (w/v) crystal violet solution. The plaques were counted by visual examination and the size of the plaques were measured by scale loupe. Virus infection and cell harvest Vero E6-ACE2 and H1299 cells were seeded in 6-well plates and allowed to attach. Cells were washed once with fresh DMEM and infected with 0.5 or 3 MOI of SARS-CoV-2 in each well. DMEM media was used as mock infection. The plates were incubated on a rocker in 33 °C for 45 min for virus adsorption. The virus inoculum was then removed and replaced by DMEM media and placed in 33 °C CO 2 incubator. The cell pellets were collected at indicated time points and stored at −80 °C. The cell pellet samples were lysed, and cell lysates were subjected to Western blot analysis or RT-qPCR for the detection of the proteins or RNA of interest. Transfection of siRNAs and plasmid DNA expression vector For siRNA knockdown, the cells were transfected with Lipofectamine RNAiMAX reagent (Thermo Fisher Scientific) with 60pmol of siRNAs (Dharmacon-GE Healthcare) according to the manufacturer’s recommendation. The control siRNA and siRNAs targeting GRP78 have been previously described [19] and their sequences are as follows: siCtrl: GAGAUCGUAUAGCAACGGUdTdT; si78#1: GGAGCGCAUUGAUACUAGAdTdT; si78#2: CUUAAGUCUCGAAUGUAAUdTdT. The construction of the expression plasmid for FLAG-GRP78 (F-GRP78) has been described previously [20] . The empty vector pcDNA3 or the expression vector for F-GRP78 was transfected into Vero E6-ACE2 and H1299 cells using the BioT Transfection Reagent (Bioland Scientific) following the manufacturer’s recommendation. The cells were incubated with the transfection mix for 48 hr before harvesting cells for immunoblot analysis of the protein of interest. Immunoblot analysis Preparation of cell lysates and immunoblot analysis has been described previously [21] . Proteins were electrophoresed in 8% or 10% SDS-PAGE gels, transferred to Nitrocellulose membrane, and probed with the following antibodies. Primary antibodies: mouse anti-GRP78 (1:1000, BD Biosciences, 610979), mouse anti-GAPDH (1:1000, Santa Cruz Biotechnology, Inc., sc-32233), mouse anti-SARS-CoV-2 Spike Protein (S1-NTD) (1:1000, Cell Signaling, #42172). Secondary antibody: mouse IgG1 binding protein conjugated to HRP (1:1000, Santa Cruz Biotechnology, Inc., sc-525408). HRP signal was detected by SuperSignal West Pico Chemiluminescence substrate (Thermo Fisher Scientific, 34080) and protein bands were visualized by ChemiDoc XRS + imager (Bio-Rad Laboratories) and quantified by Image Lab software version 4.0.1 build 6 (Bio-Rad Laboratories). RNA extraction and reverse transcription quantitative real-time PCR Vero E6-ACE2 cells were mocked infected or infected with SARS-CoV-2 at 0.5 or 3 MOI for 12 or 24 hours. The cells were lysed with TRI reagent (Millipore-Sigma, Burlington, MA) and total RNA was extracted according to the manufacturer’s recommendations. 1 μg of total RNA was used to synthesized cDNA using the qScript cDNA Supermix (QuantaBio, Beverly, MA) following manufacturer’s protocol. Quantitative real-time PCR analysis of GRP78 and GAPDH mRNA was conducted using the KAPA SYBR FAST qPCR Master Mix (Roche Sequencing and Life Science, Wilmington, MA) and analyzed by the Stratagene MX3000P Real-Time QPCR System (Agilent, Santa Clara, CA). The PCR conditions are 40 cycles, 15 s at 95 °C, 15 s at 60 °C, 15 s at 72 °C. The sequences for the primers used in this study are as followed: GRP78 5′-GTCAGGCGATTCTGGTCATT-3′ and 5′-GGTGAAAGACCCCTGACAAA-3′, GAPDH 5′- TGCACCACCAACTGCTTAGC-3′ and 5′-GGCATGGACTGTGGTCATGAG-3′. WST-1 cell viability assay Vero E6-ACE2 cells were seeded at a density of 10,000 cells per wells in a 96-well plate with DMEM media containing 10% FBS and 1% pen/strep. The cells were allowed to attached overnight and next day the media was removed and replaced with DMEM media containing 1% pen/strep and no FBS. The cells were then treated with DMSO or increasing concentrations of HA15 (0.625 μM to 5 μM). Cell viability was measured at 24, 48, and 72 hr post drug treatment using the (4-[3-(4-Iodophenyl)-2-(4-nitro-phenyl)-2H-5-tetrazolio]-1,3-benzene sulfonate) WST-1 cell proliferation assay kit (Takara Bio USA, Inc., San Jose, CA) according to manufacturer’s recommendation. Colorimetric measurement was detected using a Model 680 Microplate Reader (Bio-Rad Laboratories, Hercules, CA) at a wavelength of 450 nm and subtracted by the reference wavelength of 650 nm. Background absorbance of blank media (DMEM 1% pen/strep) was also measured and subtracted from the sample reading. Animals and in vivo procedures K18-hACE2 transgenic mice were purchased from Jackson Laboratory (cat. no. 034860). Female mice (about 10-week-old) were used. All animal care and experiments were performed according to the NIH guidelines for the care and use of laboratory animals. All animal studies were approved by the Institutional Animal Care and Use Committee of USC. Mice ( n = 3 for each group) were intranasally infected with 10 3 pfu of SARS-CoV-2 virus (USA-WA1/2020) plaque isolate in 30 μl PBS. HA15 (Cat. #CS-5825) was obtained from ChemScene (Monmouth Junction, NJ, USA). HA15 was first dissolved in DMSO and diluted in PBS for intraperitoneal injection. HA15 was intraperitoneally injected daily at 35 mg/kg from the time infected to day 3 post infection. On day 3, mice were euthanized by isoflurane overdose and the lung tissues were collected, homogenized, and lysed in 500 μl of TRIzol for RNA isolation and RT-qPCR analysis. RNA extraction and RT-qPCR analysis of mouse lung tissues Total RNA was isolated from single-cell suspended mouse tissue in 500 μl of Trizol (Thermo Fisher Scientific, Waltham, MA). RNA was extracted following the manufacturer’s protocol for the Monarch Total RNA miniprep kit (New England Biolabs, Ipswich, MA). Complementary DNA (cDNA) was generated using 100 ng of total RNA with the iScript Reverse Transcription Supermix (Bio-Rad Laboratories) following the manufacturer’s protocol. qPCR was performed in a 96-well plate with PrimeTime® Gene Expression Master Mix (Integrated DNA Technologies (IDT), Coralville, IA) in triplicate with 1 μl of cDNA using primers for SARS-CoV-2 N1 protein and murine β-actin on the Bio-Rad CFX96 Real-Time PCR Detection system. Relative gene expression of SARS-CoV-2 N protein was calculated based on a genomic equivalent (GE) standard curve using the 2019-nCoV_N_Positive Control DNA (catalog# 10006625, IDT). The GE from the experimental samples was derived from this curve using the Maestro analysis software. Pre-designed TaqMan probes were purchased from IDT: N1 [SARS-CoV-2 (2019-nCoV) CDC RUO Primers and Probes Cat# 10006713], murine β-actin (Cat# Mm.PT.39a.22214843.g). Statistical analysis All pair-wise comparisons were made using the two-tailed unpaired Student’s t test in Microsoft Excel. Data are presented as the mean ± Standard Error of the mean (S.E.M.). A p value of ≤0.05 is considered statistically significant. All graphs were generated with GraphPad Prism v.8.3.0 (GraphPad Software, San Diego, CA). Reporting summary Further information on research design is available in the Nature Research Reporting Summary linked to this article.